Mapping the evolving strain field during continental breakup from crustal anisotropy in the Afar Depression Rifting of the continents leading to plate rupture occurs by a combination of mechanical deformation and magma intrusion, yet the spatial and temporal scales over which these alternate mechanisms localize extensional strain remain controversial. Here we quantify anisotropy of the upper crust across the volcanically active Afar Triple Junction using shear-wave splitting from local earthquakes to evaluate the distribution and orientation of strain in a region of continental breakup. The pattern of S-wave splitting in Afar is best explained by anisotropy from deformation-related structures, with the dramatic change in splitting parameters into the rift axis from the increased density of dyke-induced faulting combined with a contribution from oriented melt pockets near volcanic centres. The lack of rift-perpendicular anisotropy in the lithosphere, and corroborating geoscientific evidence of extension dominated by dyking, provide strong evidence that magma intrusion achieves the majority of plate opening in this zone of incipient plate rupture. The breakup of continents and subsequent formation of new ocean basins is a fundamental component of plate tectonics that has shaped the geological record and distribution of natural resources along rifted continental margins worldwide. Continental rifts are initially characterized by relatively broad zones of mechanical extension, in which faulting and stretching of the tectonic plate accommodates strain and defines the primary architecture of the rift zone during and after rifting [1] . Ultimately, however, the locus of strain must shift towards a narrowing zone that becomes the newly formed seafloor-spreading centre [2] . It is here that magma formed from decompression melting of the mantle intrudes the plate and creates new ocean floor [3] . Despite the importance of continental breakup in plate tectonic theory, the spatial and temporal scales over which these alternate mechanisms localize strain remains controversial [2] , [4] . Lithospheric extension results in the formation of anisotropic fabrics that can be measured using seismic methods [5] , [6] , and therefore constraining the type, magnitude and orientation of seismic anisotropy over a range of depths and length scales provide a powerful tool to evaluate rifting processes [5] , [6] , [7] , [8] , [9] . Here, we quantify anisotropy of the upper crust across the seismically [10] and volcanically [11] active Afar Triple Junction using shear-wave splitting from local earthquakes to evaluate the evolving strain field in a region of incipient continental breakup [12] . The region comprises the three rift arms of the Afar Triple Junction that formed during the past ∼ 30 Myrs from the rifting of Africa and Arabia within a Paleogene flood basalt province [13] ( Fig. 1 ). The topographic depression is flanked by large offset, seismically active border faults initially formed during plate stretching in Oligo-Miocene times [14] . Since <4 Myr ago, however, volcanism and dyke-induced normal faulting have localized to ∼ 15-km-wide, ∼ 60-km-long axial volcanic ranges with aligned chains of basaltic cones and fissural flows [12] , [15] . These Quaternary-Recent magmatic segments (for example, Dabbahu segment) are similar in size, morphology, structure and spacing to the second-order ( ∼ 50 km-long) non-transform segments of a slow-spreading mid-ocean ridge [12] , [15] ( Fig. 1 ). The highly extended and intruded crust beneath most of the Afar Depression is ∼ 18–25 km thick, contrasting the ∼ 35–45-km-thick crust of the relatively unfaulted adjacent plateaux [16] . Kinematic models constrained by Global Positioning System (GPS) data suggest ∼ 5 mm per year of ∼ N100°E opening occurs in the Main Ethiopian rift (MER) [17] , [19] and ∼ 20 mm per year of ∼ N50°E extension across the Red Sea rift (RSR) [18] , [19] ( Fig. 1 ). Structural data [14] and kinematic models based on geodetic data [19] suggest the Quaternary-Recent magmatic segments of the MER extend as far north as the Tendaho-Goba'ad Discontinuity (TGD; Fig. 1 ). Rifting in Ethiopia currently occurs above a broad, slow seismic velocity anomaly in the mantle, interpreted as a region of anomalously high temperature and partial melt that is caused primarily by the combined effects of the African superswell and ongoing lithospheric thinning [20] , [21] . 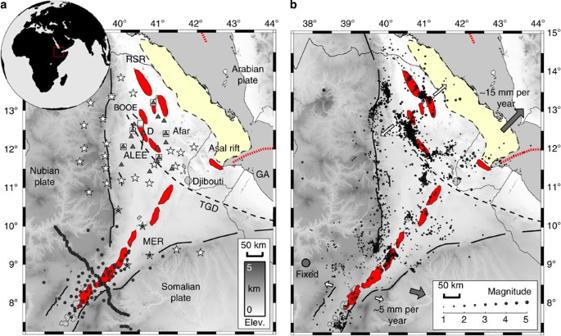Figure 1: Distribution of seismic stations and earthquakes in Ethiopia during 2001–2009. (a) Temporary seismic stations deployed in Ethiopia plotted on SRTM digital elevation model. Grey circles are from the Ethiopia Afar Geoscientific Lithospheric Experiment (EAGLE) during October 2001–February 2003. White squares are from the Boina Broadband Network operational during October 2005–September 2006. Grey triangles are 'SEARIFT' seismic stations operating during March 2007–October 2009. White stars are 'Afar Consortium' seismic stations deployed during October 2007–October 2009. BOOE and ALEE are seismic stations Boina and Ado'Ale, respectively, deployed in the Dabbahu magmatic segment (D). Solid black lines are Oligo-Miocene age border faults. Solid red shapes are Quaternary-Recent magmatic segments. The Main Ethiopian rift (MER), Red Sea rift (RSR) and Gulf of Aden (GA) rift form the three arms of the Afar Triple Junction. Dashed-red lines show zones of submarine seafloor spreading. The MER terminates at the Tendaho-Goba'ad Discontinuity (TGD), shown by a black dashed line. (b) Distribution of local seismicity recorded during the operation of the named temporary seismic stations. Motions of the Arabian and Somalian plates relative to a fixed Nubian plate are shown as grey arrows. Figure 1: Distribution of seismic stations and earthquakes in Ethiopia during 2001–2009. ( a ) Temporary seismic stations deployed in Ethiopia plotted on SRTM digital elevation model. Grey circles are from the Ethiopia Afar Geoscientific Lithospheric Experiment (EAGLE) during October 2001–February 2003. White squares are from the Boina Broadband Network operational during October 2005–September 2006. Grey triangles are 'SEARIFT' seismic stations operating during March 2007–October 2009. White stars are 'Afar Consortium' seismic stations deployed during October 2007–October 2009. BOOE and ALEE are seismic stations Boina and Ado'Ale, respectively, deployed in the Dabbahu magmatic segment (D). Solid black lines are Oligo-Miocene age border faults. Solid red shapes are Quaternary-Recent magmatic segments. The Main Ethiopian rift (MER), Red Sea rift (RSR) and Gulf of Aden (GA) rift form the three arms of the Afar Triple Junction. Dashed-red lines show zones of submarine seafloor spreading. The MER terminates at the Tendaho-Goba'ad Discontinuity (TGD), shown by a black dashed line. ( b ) Distribution of local seismicity recorded during the operation of the named temporary seismic stations. Motions of the Arabian and Somalian plates relative to a fixed Nubian plate are shown as grey arrows. Full size image We present analysis of S-wave splitting in Afar and show that it is best explained by anisotropy from strain-related structures, with the dramatic change in splitting parameters into the rift axis from the increased density of dyke-induced faulting combined with a contribution from oriented melt pockets near volcanic centres. The lack of rift-perpendicular anisotropy in the lithosphere, and corroborating geological and geophysical evidence of strain dominated by dyking, provide strong evidence that localized magma intrusion accommodates the majority of plate opening in this zone of magma-rich plate rupture, without slip along detachment faults. Quantifying anisotropy from S-wave splitting measurements We conduct S-wave splitting analysis on 78 seismograms from 34 seismic stations in Ethiopia to constrain the polarization direction of the fast S-wave ( φ ) and the time delay between the fast and slow S-waves (δ t ) ( Supplementary Fig. S1 ). The seismograms are derived from local earthquakes in Ethiopia occurring at a depth of 4–22 km ( Supplementary Table S1 ). More than one S-wave splitting measurement is available at a number of the seismic stations ( Fig. 2 ). In these cases, δt increases nearly linearly with ray-path distance between the hypocentre and seismic station, a pattern most clearly seen for the 6 splitting measurements at BOOE and for the 30 splitting measurements at ALEE ( Fig. 2 , Supplementary Figs S2 and S3 ). This strongly suggests that S-wave splitting is incrementally accrued along the full ray-path length, and we therefore normalize δt measurements by deriving percent (%) S-wave anisotropy beneath each station assuming uniformly distributed anisotropy through the crust. In addition, the 30 measurements from station ALEE have sufficient range in backazimuth to allow us to invert the data set for fractures parameters [22] . The splitting parameters are best-fit by a simple homogeneous fracture-induced model with a fracture strike of 145±10° and fracture density of 0.063±0.015 ( Supplementary Fig. S4 ). At ALEE, the average φ and percent anisotropy are 147° and 5%, respectively. For the other stations with more than one splitting measurement, φ shows little variation between measurements, and we therefore plot and interpret the average measured fast direction with the 2-sigma error estimate within ±12° ( Fig. 3 , Supplementary Table S2 ). We see no evidence for temporal changes in splitting parameters at any of our stations as seen near active volcanoes with shallow magma chambers elsewhere [23] , [24] ( Supplementary Fig. S3 ). 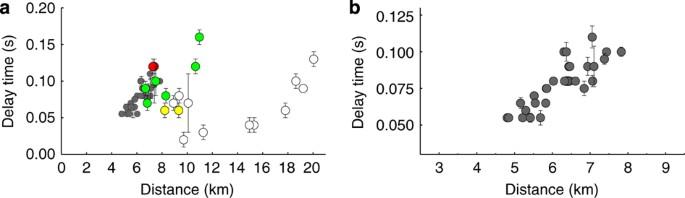Figure 2: Variation in splitting delay time versus distance travelled by the seismic wave. Individual shear-wave splitting delay times (δt) are plotted versus ray-path distance between the hypocentre and seismic station for the Afar region. White circles show all the stations at which only one splitting measurement is available. Coloured circles show seismic stations from which more than one splitting is available, with each colour denoting a different station. Red measurements are from SRDE and yellow measurements are from KOBE. Green measurements are from BOOE and grey measurements are from ALEE. (a) All new measurements made in this study, and (b) measurements from station ALEE only. Station locations are shown inFigure 1. Figure 2: Variation in splitting delay time versus distance travelled by the seismic wave. Individual shear-wave splitting delay times (δ t ) are plotted versus ray-path distance between the hypocentre and seismic station for the Afar region. White circles show all the stations at which only one splitting measurement is available. Coloured circles show seismic stations from which more than one splitting is available, with each colour denoting a different station. Red measurements are from SRDE and yellow measurements are from KOBE. Green measurements are from BOOE and grey measurements are from ALEE. ( a ) All new measurements made in this study, and ( b ) measurements from station ALEE only. Station locations are shown in Figure 1 . 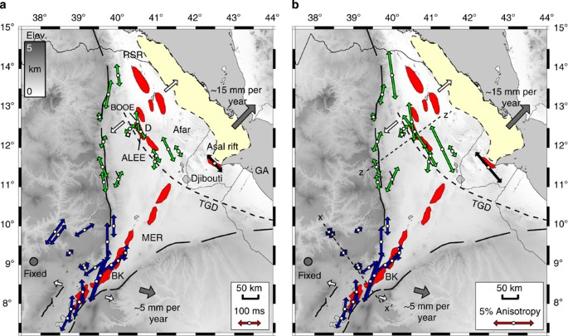Figure 3: Orientation and magnitude of crustal shear-wave splitting measurements in the Ethiopian and Afar rifts. (a) Local earthquake shear-wave splitting measurements in Ethiopia. The arrows are oriented parallel to the fast-polarization direction (φ) and the arrow length is scaled by delay time (δt). Measurements from Keiret al.25from the MER are in blue, and an average of measurements from the Asal rift in Djibouti are black. New splitting measurements from our study are green. (b) Estimate of magnitude and direction of anisotropy derived from the raw S-wave splitting measurements displayed ina. The arrows are oriented parallel to the fast anisotropic direction and the arrow lengths are scaled to % anisotropy, assuming that S-wave splitting is accrued along the full ray-path length. In the MER, crustal anisotropy is particularly high and in the Boset-Kone (BK) magmatic segment where Quaternary-Recent volcanism is particularly voluminous. The profiles displayed inFigure 4arex–x′ andz–z′. Full size image Figure 3: Orientation and magnitude of crustal shear-wave splitting measurements in the Ethiopian and Afar rifts. ( a ) Local earthquake shear-wave splitting measurements in Ethiopia. The arrows are oriented parallel to the fast-polarization direction ( φ ) and the arrow length is scaled by delay time (δ t ). Measurements from Keir et al . [25] from the MER are in blue, and an average of measurements from the Asal rift in Djibouti are black. New splitting measurements from our study are green. ( b ) Estimate of magnitude and direction of anisotropy derived from the raw S-wave splitting measurements displayed in a . The arrows are oriented parallel to the fast anisotropic direction and the arrow lengths are scaled to % anisotropy, assuming that S-wave splitting is accrued along the full ray-path length. In the MER, crustal anisotropy is particularly high and in the Boset-Kone (BK) magmatic segment where Quaternary-Recent volcanism is particularly voluminous. 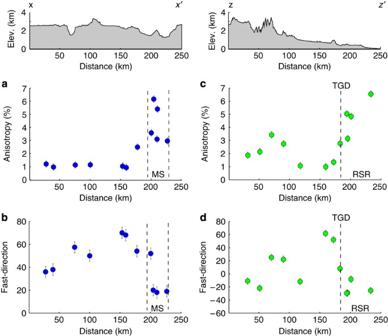Figure 4: Profiles of shear-wave splitting parameters across the rift valleys in Ethiopia. The across-rift profiles show variation in splitting parameters at stations located 100 km either side of profilesx–x′ for the MER andz–z′ across Afar. For both the MER (a,b) and RSR (c,d), note the dramatic increase in magnitude of anisotropy synchronous with rotation of fast direction into the Quaternary-Recent magmatic segments. The top two panels show topography along the displayed profiles. The profiles displayed in Figure 4 are x – x ′ and z – z ′. Full size image Crustal anisotropy of the Afar Depression Our S-wave splitting measurements from local earthquakes in Afar show large spatial variations in both φ and δ t that correlate to major tectonic structures in the region ( Fig. 3a ). At stations along the western margin of Afar, φ is oriented ∼ NNW (North-Northwest) to NNE (North-Northeast), sub-parallel to the orientation of the Oligo-Miocene border faults. δ t is 0.04–0.13 s for earthquakes that are 4–15 km deep, equivalent to 1–2.8% anisotropy ( Fig. 3 ). At stations within the Afar Depression and west of the TGD, φ is oriented ∼ NNE to ∼ NE (Northeast), and δ t is 0.04–0.07 s for earthquakes that are 5–10 km deep, also equating to 1–2.8% anisotropy ( Fig. 3 ). These measurements contrast with those made at stations located near Quaternary-Recent magmatic segments east of the TGD, where φ is oriented at ∼ NW (Northwest) to ∼ NNW, parallel to aligned cones, fissures and faults observed at the surface. Delay times from these stations are 0.04–0.12 s for earthquakes that are just 5–8 km deep, which equates to a larger magnitude of anisotropy of up to 6.5% ( Fig. 3 ). Crustal anisotropy of the Main Ethiopian Rift Further south near the MER, S-wave splitting measurements are available from the interior of the NW plateau, on the western rift margin, and from the Quaternary-Recent magmatic segments within the rift ( Fig. 3 ). At stations on the NW plateau φ strikes ∼ NE–ENE (East-Northeast). δt is relatively low at between 0.04 s and 0.14 s for earthquakes at depths of 12–20 km, equating to spatially uniform anisotropy of just 1.1% (ref. 25 ). Near the MER border faults, δ t is 0.1–0.16 s, which is 2.2–3.6% anisotropy. φ varies between ∼ N and ∼ NE, spatially correlating with the change in strike of the Oligo-Miocene border faults as the MER opens into the Afar Depression. At stations near the Quaternary-Recent magmatic segments, φ is mostly oriented ∼ N to NNE, again parallel to the orientation of Quaternary-Recent structures. Here, delay times are 0.06–0.24 s for earthquakes that are just 6–9 km deep, equating to 3–6.2% anisotropy ( Fig. 3 ). Anisotropy of the upper crust is commonly attributed to dilatancy of micro-cracks generating a fast-polarization direction perpendicular to the minimum horizontal stress (SHmin) [26] . Such stress-induced anisotropy is most pronounced nearest the surface and the effect decreases with depth as the confining pressure increases, causing micro-cracks to close [27] . A model of stress-induced crack anisotropy successfully explains observations of temporal changes in fast directions. For example, φ at active volcanoes are usually parallel to the regional SHmin, with 90° polarization flips observed before volcanic eruption interpreted as caused by a change in crack orientation induced by magma reservoir inflation [23] . Alternatively, anisotropy in the crust can also be caused by strain-induced Earth structures such as aligned macro-scale fractures and faults related to regional tectonics, fault-zone fabrics and aligned minerals and/or grains [6] , [28] , which cause the S-waves to be polarized with the fast direction in the plane of the feature. The presence of aligned melt within magmatic structures such as dykes, commonly used to explain patterns of mantle anisotropy in magma-rich extensional settings [5] , [29] , also provides an efficient means of generating seismic anisotropy in the crust [30] , [31] . Discriminating stress-induced and structure-induced anisotropy is relatively simple in regions where dominant structures are oblique to SHmin, using measurements of φ [28] , but can be more challenging in regions where structural features align perpendicular to SHmin. In Ethiopia, the orientation of the fast S-wave universally parallels the strike of dominant Earth structures, and is not always perpendicular to SHmin inferred from current rift opening. This, combined with evidence that anisotropy is relatively evenly distributed with depth ( Fig. 2 ) and the lack of temporal variations in splitting parameters, suggest that structure-induced anisotropy dominates the upper crust beneath the region. Such a pattern is clear along the margins of the MER and Afar, where φ is parallel to Oligo-Miocene border faults but not perpendicular to the direction of extension. Similarly in the interior of the plateau, φ is ∼ NE to ∼ ENE, a 45° obliquity to the ∼ ESE (East-Southeast) directed-extension across the MER ( Fig. 3 ). Beneath the plateau and away from extensional structures associated with rifting, splitting likely parallels pre-existing metamorphic basement foliation [25] . In the Quaternary-Recent magmatic segments of the MER and Afar, the dominant strike of extensional features such as faults and aligned cones is perpendicular to rift-opening direction [32] , [33] , [34] , resulting in observed φ that is perpendicular to the inferred SHmin. At stations in the MER, φ varies between ∼ N–NE, with a modal strike of ∼ NNE, orthogonal to the ∼ N105°E extension direction ( Figs 3 and 4 ). In Afar, at stations east of the TGD and therefore in the Gulf of Aden and RSRs, φ is ∼ NNW–NW, approximately parallel to the strike of faults and aligned volcanic cones here, and orthogonal to the direction of extension ( Figs 3 and 4 ). We observe a systematic clockwise rotation of φ from ∼ NW in the Asal rift of Djibouti to ∼ NNW in northern Afar, a rotation that closely mimics along-strike variation in rift opening determined using GPS measurements [19] . A striking feature in the data is the marked similarity between φ and the strike of elongate clusters of seismicity in the three rifts of the Afar triple junction ( Fig. 1b ). This, along with MER parallel ∼ NE-NNE oriented φ at stations located within Afar but west of the TGD lend support to structural measurements [14] and kinematic models [19] that suggest the TGD currently partitions most extension related to the separation of the Arabian Plate from Africa, and that between the Somalian and Nubian Plates in the East African rift. Figure 4: Profiles of shear-wave splitting parameters across the rift valleys in Ethiopia. The across-rift profiles show variation in splitting parameters at stations located 100 km either side of profiles x – x ′ for the MER and z – z ′ across Afar. For both the MER ( a , b ) and RSR ( c , d ), note the dramatic increase in magnitude of anisotropy synchronous with rotation of fast direction into the Quaternary-Recent magmatic segments. The top two panels show topography along the displayed profiles. Full size image The sensitivity of crustal anisotropy in the region to ongoing rifting processes is further supported by the increase in magnitude of anisotropy in zones of Quaternary-Recent strain localization ( Figs 3b and 4 ). Stations near the axial magmatic segments show anisotropy of up to 6.5%, whereas regions on the margins of the rift valley and adjacent plateau exhibit a lower magnitude of anisotropy ( Figs 3b and 4 ). As we observe an increase in degree of surface fissuring and dyke-induced faulting into the rift axis [35] , [36] , an increased density of macroscopic fractures and faults in the upper crust provides the simplest model to explain the pattern of S-wave splitting. However, the increase in degree of anisotropy into the magmatic segments is also concomitant with the presence of Quaternary-Recent magmatism, suggesting a link between anisotropy and ongoing magmatic processes. Along-axis variations in magnitude of anisotropy commonly correlate to volcanic productivity. In the MER for example, anisotropy is high ( ∼ 6%) at stations located on volcanoes in the Boset-Kone magmatic segment, where surface fracturing is minimal and the volume of Quaternary-Recent eruptions is locally high [37] . The preferred alignment of melt inclusions (oriented melt pockets) is a very effective way to generate anisotropy [38] , with the magnitude of anisotropy sensitive to the volume fraction of the melt and shape of the melt inclusions [39] . Direct constraints on geometry of aligned melt come from combined geodetic and seismic observations of active dyking beneath the Dabbahu segment in the Afar rift. In general, these dykes are ∼ 1–8 m wide, ∼ 10–30 km long and therefore have aspect ratios of <0.001 (refs 40 , 41 , 42 , 43 ), a geometry most effective for generating seismic anisotropy [38] , [39] . In the MER, a model of oriented melt pocket-induced anisotropy in the upper 90 km (lower crust, lithospheric mantle and upper asthenosphere) including just 0.1% partial melt is required to explain the spatial variations in SKS splitting [5] , [44] . In addition, the azimuthal variation in the propagation of surface waves in the MER shows that oriented melt pockets is also the dominant mechanism of seismic anisotropy in the lower crust and mantle lithosphere ( ∼ 20–50 km) [31] . At this depth range, Quaternary xenolith bearing basalts show that partial melts reside in dykes/veins intruded into the plate beneath the Quaternary-Recent magmatic segments [45] . In the lithospheric mantle and lower crust beneath Ethiopia, we do not see the rift-perpendicular anisotropy expected from stretching-induced crystal alignment that commonly characterizes other regions of extension with little magmatism such as the western United States [6] . It is likely that early stretching-induced anisotropy has been largely overprinted by later rift-parallel dyking into the plate, and/or that anisotropy due to rift-parallel dyking dominates the anisotropy induced by synchronous stretching and associated thinning of the intruded plate. Indeed, in the northernmost ∼ 100 km of the Afar Depression, the close association between marked Pliocene-Recent subsidence of the land towards and below sea-level and the presence of thinner (<15-km-thick) crust suggests stretching and volcanic loading of the intruded Afar plate occurs just before the onset of seafloor spreading [46] . The applicability of oriented melt pocket dominated anisotropy in the upper crust near active volcanic centres in the Quaternary-Recent magmatic segments is appealing, and supported by geodetic observations of volcano deformation showing modern examples of more than a year-long recharge of shallow magmatic plumbing systems in the MER, RSR and Gulf of Aden [47] . This shallow magma causes high seismic attenuation and scattering in the upper crust beneath volcanoes [48] . Residence of partial melts at shallow depths is further supported by the petrology of Quaternary lavas from axial volcanoes showing rift axial magmas predominantly fractionate in upper crustal plumbing systems [49] . In the axial magmatic segments, but away from eruptive centres, approximately metres-wide basaltic dykes injected laterally into the upper crust likely freeze within day to week-long timescales after emplacement, and therefore are unlikely to contribute to oriented melt pocket-induced anisotropy. Instead, the large magnitude of rift-parallel anisotropy in the rift axis away from volcanic centres is best explained by high density of dyke-induced fracturing and faulting. Anisotropy of the upper crust derived from S-wave splitting of local earthquakes maps out the strain field around the three rifting arms of the Afar Triple Junction. An increase in density of dyke-induced fracturing and faulting into the zones of localized Quaternary-Recent magma intrusion, combined with a contribution from oriented melt pockets near active magmatic centres best explains the increase in magnitude of anisotropy into the rift axis and concomitant rotation of the fast S-wave to rift parallel directions. Our observations and corroborating geological and geophysical data from the ongoing Dabbahu rifting episode in Afar, provide strong evidence that localized dike intrusion and shallow faulting above the dike accommodates the majority of plate opening, with little evidence for strain accommodated by detachment faulting as seen on magma-poor margins [50] . Local earthquake data sets in Ethiopia We present a total of 78 S-wave splitting measurements at 34 seismic stations in Ethiopia, derived from local earthquakes at a depth of 4–22 km. These data were recorded during 2001–2009 by six temporary networks of broadband seismic stations. Measurements from the MER are derived from the study of Keir et al . from EAGLE 1, 2 and 3 broadband networks that recorded local seismicity during October 2001 to January 2003 (refs 25 , 51 ). New shear-wave splitting measurements presented here in the Afar Depression and adjacent Ethiopian Plateau are made on local earthquakes recorded during 2005–2009 by three temporary networks of broadband seismic stations. From October 2005 to November 2006, ∼ 2,000 local earthquakes were located from seismic data recorded on the 'Boina Broadband Network', consisting of up to nine Güralp 6TD seismometers in northern Afar ( Fig. 1 ) [41] , [52] . These data yield seven S-wave splitting measurements at two seismic stations. The majority of data for our study is from the 'SEARIFT' network comprising up to 16 Güralp 40TD seismometers in northern and central Afar during March 2007–October 2009, and the 'Afar Consortium Experiment' network comprising 1 Güralp 6TD, 23 Güralp ESP and 3 Güralp 3T seismometers in Afar and on the adjacent uplifted plateaux during October 2007–October 2009 ( Fig. 1 ) [42] , [53] . Stations from these two temporally overlapping networks recorded ∼ 5,300 local earthquakes ( Fig. 1 ), on which 45 S-wave splitting measurements could be obtained at 14 seismic stations. All seismic stations recorded data at a sampling frequency of 50 Hz. We also interpret published S-wave splitting measurements from the Asal-Ghoubbet rift in Djibouti [54] ( Fig. 3 ). Details of techniques used to locate earthquakes and associated errors are available in the seismicity studies by Keir et al . [55] for the MER, Ebinger et al . [52] and Belachew et al . [53] for the Afar region, and Lépine and Hirn [54] in Djibouti. However, for all these studies the error in depth of earthquakes located within the S-wave window is estimated at less than ±1 km in both depth and horizontal position. Shear-wave splitting measurements The polarization direction of the fast S-wave ( φ ) and the time delay between the fast and slow S-waves (δt) is determined using the method of Silver and Chan [56] , adapted for application to micro-earthquakes. In an isotropic radially stratified crust, near vertically impinging S-waves should exhibit linear particle motion. However, this phase is split into orthogonally polarized fast and slow S-waves when it travels through an anisotropic medium, producing an elliptical particle motion and energy on the transverse component seismogram. The splitting can be quantified by the time delay between the two S-waves (δ t ) and the orientation of the fast S-wave ( φ ). To remove the effects of the anisotropy, we rotate the horizontal components by φ and shift their relative positions by δ t to minimize the second eigen value of the covariance matrix for particle motion of a time window around the S-wave arrival, thereby linearizing the particle motion. To estimate the splitting, we perform a grid search for the correction parameters that best linearize the S-wave motion. Splitting measurements are made for 100 different time windows selected around the S-wave. Cluster analysis is then used to find the most suitable splitting parameters [57] . An F-test is performed to assess the uniqueness of the estimated splitting parameters and thereby produce an error estimate [58] . The splitting parameters are well constrained. We use a cut off error criteria of ±0.04 s for δ t and 12° for φ ( Supplementary Table S1 ). An example of this analysis is shown in Supplementary Figure S1 . We are restricted to using three-component seismograms where the S-wave incidence-angle is within the shear-wave window (SWW). The SWW is the vertical cone bound by sin −1 ( V s/ V p), where S-wave particle motions are not disturbed by S–P conversions at the free surface [59] . We use a V p/ V s of 1.75, calculated from P- and S-wave travel-times from earthquakes in the MER and Afar, which corresponds to a SWW that is a cone within 35 o of the vertical. For hypocentres within the SWW of available stations, we restrict measurements to sharp S-wave arrivals with a high signal to noise ratio and band-pass filter the data at 1–7 Hz, as the S-waves in our study typically have a characteristic period of 4 Hz. The selection criterion severely limit the number of earthquakes on which S-wave splitting measurements can be made in a region in which seismicity is most commonly located outside the S-wave window. Modelling fracture properties The 30 S-wave splitting measurements from station ALEE, located within the Dabbahu magmatic segment, have sufficient range in backazimuth to allow us to invert the data set for best-fit density and strike of fractures. At face value, the splitting parameters for these earthquakes show a systematic trend with distance (latitude) along the segment ( Supplementary Figs S2 and S3 ). The fast S-wave polarization ( φ ) rotates smoothly from 115° in the north to 165° in the south, suggesting a rotation in the dominant fracture pattern. Similarly, the delay time (δ t ) decreases from over 0.10 s to 0.05 s, suggesting a decrease in fracture density towards the south. However, this interpretation of these observations neglects variations due to the changing azimuth and inclination of the ray paths. Most studies of S-wave splitting use phases with near-vertical ray paths beneath the receiver (for example, SKS). However, in any anisotropic model splitting parameters will vary with both azimuth and slowness (angle of inclination). For example, rays propagating perpendicular to the plane of fractures will not show any splitting (a null direction), whereas rays propagating parallel to the fractures will show maximum S-wave splitting. All events recorded at station ALEE are within the S-wave window, but nevertheless show variation in slowness and azimuth. A simple homogeneous fracture-induced model can explain the spatial variations in observed splitting parameters. Verdon et al . (2009) show how simple rock physics models can be used to guide inversions of S-wave splitting measurements to obtain estimates of fracture parameters [22] ( Supplementary Fig. S4 ). Here we assume that the anisotropy is due to a combination of an aligned vertical fracture set superimposed on a vertically transversely isotropic (VTI) material. The VTI anisotropy can be explained by the rhythmical layering of volcanic rocks and sediments in the upper 5–10 km of crust, as noted by Kendall et al . [60] and Bastow et al . [31] Using the inversion scheme of Verdon et al ., [22] we estimate the fracture strike to be 145±10° and a fracture density of 0.063±0.015 ( Supplementary Fig. S4 ). The strike of fractures is consistent with orientation of fractures mapped on the surface ( Supplementary Fig. S5 ). We can also estimate two of the three Thomsen parameters that describe VTI anisotropy (gamma and delta). However, neither of these parameters are well constrained, because of the lack of horizontally propagating rays. We instead fix the VTI parameters to gamma=0.05 and delta=0.05, which is broadly in line with the estimates of Bastow et al . for anisotropy in the shallow crust in the MER [31] . We note that our estimates of fracture strike and density are not very sensitive to the choice of VTI parameters. We also tried inverting for a conjugate set of fractures, but this analysis confirmed that only a single set with a strike of roughly 145° and a fracture density of roughly 0.06 is required. How to cite this article: Keir, D. et al . Mapping the evolving strain field during continental breakup from crustal anisotropy in the Afar Depression. Nat. Commun. 2:285 doi: 10.1038/ncomms1287 (2011).